Fumigant methyl iodide can methylate inorganic mercury species in natural waters Methyl iodide or iodomethane (CH 3 I) has recently been registered as a fumigant in many countries, although its environmental impacts are not well understood. Here we report the results of a study on the methylation of mercury by CH 3 I in natural water by incubation experiments using both Hg ( 199 HgCl 2 and )- and hydrogen (CD 3 I)-stable isotope addition techniques. We find that methylation of Hg 0 , and Hg 2+ by CH 3 I can occur in natural water under sunlight, while only Hg 0 and can be methylated in deionized water. We propose that the methylation of Hg by CH 3 I in natural waters is mediated by sunlight and involves two steps, the reduction of Hg 2+ to Hg 0 / and the subsequent methylation of Hg 0 / by CH 3 I. Further quantitative assessment suggests that CH 3 I-involved methylation of inorganic Hg could be an important source of CH 3 Hg + in an environment where CH 3 I has been used in large amounts as a fumigant. Methyl iodide or iodomethane (CH 3 I) is one of the most abundant organoiodine compounds in natural environments [1] . Anthropogenic input of CH 3 I to the environment has been rapidly increasing since the 1990s, after it was suggested as a replacement for the ozone-depleting fumigant methyl bromide (CH 3 Br). CH 3 I is preferred over CH 3 Br because it is similar to, or more effective than, CH 3 Br in controlling a wide variety of soil pests and weeds [2] , and it has less impact on the ozone layer owing to its rapid photodegradation in the troposphere [2] . The U.S. EPA approved the use of CH 3 I as a fumigant in 2008 (ref. 3 ). A commercially available CH 3 I formulation was then registered in many countries, such as the USA, Japan and New Zealand. The potentially negative impact of using CH 3 I has not been adequately addressed [4] , despite its increasing use on farmland. Compared with CH 3 Br, CH 3 I degrades more slowly in soil, hence increasing its chance of being transported to an aquatic environment via runoff [5] , [6] . CH 3 I is known to have the capability of methylating several metals and metalloids, including Sn 2+ , As 3+ , Pb 2+ and Hg 0 , following an oxidative addition mechanism [7] , [8] , [9] , [10] . Among these metals/metalloids, mercury deserves special attention because its methylation product, methylmercury (CH 3 Hg + ), is among the most widespread of all highly toxic contaminants. Previous work has demonstrated that CH 3 I can be used as a methylation reagent for synthesizing CH 3 Hg + from Hg 0 in a laboratory setting [10] . However, such a methylation reaction has not been confirmed in natural waters with low concentrations of Hg 0 and CH 3 I (ref. 11 ). The undetectable CH 3 Hg + in the previous study could be attributed to the possible degradation of CH 3 Hg + , which was not monitored during the experiment [11] . It is understandable that direct methylation of Hg 2+ by CH 3 I has not been observed [12] , [13] , [14] , as this reaction is theoretically impossible according to the mechanism of the oxidative addition reaction. However, recent studies have indicated that a rapid conversion of Hg 2+ to Hg 0 can occur in natural waters [15] , [16] , suggesting that Hg 2+ could also play an important role in the CH 3 I-involved methylation of inorganic mercury in the environment. In this study, we show that CH 3 I has the potential of methylating inorganic mercury in aquatic environments under sunlight. We used both mercury ( 199 HgCl 2 and )- and hydrogen (CD 3 I)-stable isotopes to examine the possible methylation of inorganic mercury species by CH 3 I in natural water. Various concentrations of 199 HgCl 2 , Hg 2 (NO 3 ) 2 , Hg 0 and CH 3 I were added to deionized water or natural water and incubated with or without sunlight. , spiked in the incubation media, was used as a control to correct for the degradation of produced CH 3 Hg + . CD 3 I was used to validate the source of the methyl group in CH 3 Hg + . Our results demonstrate that methylation of inorganic mercury by CH 3 I could be an important source of CH 3 Hg + in CH 3 I-contaminated surface water. Methylation of inorganic mercury by CH 3 I in natural water Natural water samples were collected from a pond located at the Florida International University (FIU). Methylation experiments were carried out in a closed 0.5-l Teflon bottle under natural sunlight or in darkness. The methylation of inorganic mercury species (Hg 2+ , and Hg 0 ) by CH 3 I was measured ( Fig. 1 ). Significant production of CH 3 Hg + was observed in waters exposed to sunlight for all tested mercury species. For samples tested in the dark, no significant formation of CH 3 Hg + occurred for Hg 2+ and Hg 0 ( P >0.1) ( Fig. 1a,c ), and a 90% reduction in the formation of CH 3 Hg + was observed for ( P <0.05) when compared with that under sunlight ( Fig. 1b ). Most previous studies also showed that sunlight is necessary for the methylation of Hg 0 by CH 3 I [10] , [11] , [17] , although contrast results were also observed [18] . In sunlight, the methylation rates of these three mercury species ( r , equation (9), see Methods) were in the order of Hg 0 (1.67±0.09 pmol l −1 E −1 m 2 )> (0.424±0.025 pmol l −1 E −1 m 2 )>Hg 2+ (0.125±0.010 pmol l −1 E −1 m 2 ). These results suggest that methylation of mercury by CH 3 I can occur in natural water and this process is driven by sunlight. The 1-day methylation yield of Hg 0 by CH 3 I was calculated to be 0.6%, comparable with the results of Celo et al . [18] , [19] and Hall et al . [11] (1.1 and 0.29%, respectively). Although methylation rates of Hg 0 and were ~13- and 4-fold higher than that of Hg 2+ , methylation of Hg 2+ by CH 3 I should be more important as Hg 2+ is the main inorganic mercury species in natural water. The formation of CH 3 199 Hg + with the addition of 199 Hg 2+ demonstrated that the generated CH 3 Hg + was from the methylation of spiked 199 Hg 2+ ( Supplementary Fig. 1a ). Further experiments were conducted to examine the origin of the methyl group of CH 3 Hg + using a CD 3 I tracer method. When natural water containing Hg 2+ was spiked with CD 3 I and incubated under sunlight for 4 days, formation of CD 3 Hg + was detected using gas chromatography–mass chromatography (GC–MS) ( Supplementary Fig. 1b ) (detailed description is given in Supplementary Note 1 ). Based on the oxidative addition theory, Hg 2+ cannot be directly methylated by CH 3 I. It is therefore proposed that the observed methylation of Hg 2+ in natural water may proceed through a two-step reaction mechanism, the reduction of Hg 2+ to Hg 0 or followed by the methylation of Hg 0 or by CH 3 I (Equations (1, 2, 3, 4, 5)). Considering the electronegativity of the iodine atom, CH 3 I is expected to dissociate to CH 3 ./I. or CH 3 + /I − , but not CH 3 − /I + (ref. 20 ). CH 3 . and CH 3 + can then methylate or Hg 0 . According to the density functional theory, the methylation reaction of Hg 0 and CH 3 I is thermodynamically favourable [17] . The requirement of sunlight for this reaction indicates the existence of a high activation barrier [17] . This proposed mechanism of Hg 2+ methylation is supported by the facts that 95.2 pmol l −1 Hg 0 was detected in the pond water spiked with 4.99 nmol l −1 Hg 2+ ( Supplementary Fig. 2 ) and that the methylation rate of Hg 2+ was only 7.5% and 29.5% compared with that of Hg 0 and ( Fig. 1 ). The formation of during Hg 2+ photoreduction in the presence of dissolved organic matter (DOM, Suwannee River humic acid) was also confirmed using Raman spectrometry ( Supplementary Fig. 3 ). These results provide strong evidences to support the proposed two-step reaction mechanism of CH 3 I-involved methylation of mercury in natural water. 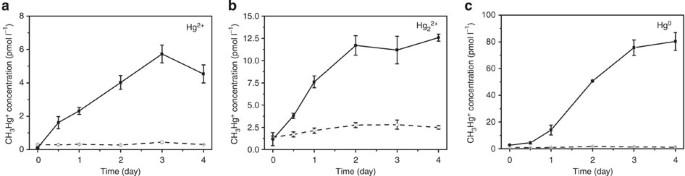Figure 1: Methylation of inorganic Hg by CH3I in pond water. (a) Hg2+, (b)and (c), Hg0. Solid line and dashed line represent the methylation of inorganic Hg under sunlight and in the dark, respectively. CH3I was spiked into the pond water to form a final concentration of 1 mmol l−1. The final concentrations of Hg2+,and Hg0were 4.99, 4.99 and 4.24 nmol l−1(as Hg), respectively. The methylation rates for Hg2+,and Hg0were calculated to be 0.125±0.010, 0.424±0.025 and 1.67±0.09 pmol l−1E−1m2, respectively. All the tests were conducted in triplicate, and the error bars indicate the s.d. of three repeated measurements. Figure 1: Methylation of inorganic Hg by CH 3 I in pond water. ( a ) Hg 2+ , ( b ) and ( c ), Hg 0 . Solid line and dashed line represent the methylation of inorganic Hg under sunlight and in the dark, respectively. CH 3 I was spiked into the pond water to form a final concentration of 1 mmol l −1 . The final concentrations of Hg 2+ , and Hg 0 were 4.99, 4.99 and 4.24 nmol l −1 (as Hg), respectively. The methylation rates for Hg 2+ , and Hg 0 were calculated to be 0.125±0.010, 0.424±0.025 and 1.67±0.09 pmol l −1 E −1 m 2 , respectively. All the tests were conducted in triplicate, and the error bars indicate the s.d. of three repeated measurements. Full size image To evaluate the importance of CH 3 Hg + formed through CH 3 I-involved process in aquatic environments, additional experiments were performed in natural waters from the Florida Everglades. In these experiments, the methylation of Hg 2+ by CH 3 I was also observed ( Supplementary Fig. 4 ), indicating that this process may widely occur in aquatic environments. Methylation rates ( r ) were calculated to be 0.025±0.001 pmol l −1 E −1 m 2 and 0.125±0.010 pmol l −1 E −1 m 2 for surface water of the Florida Everglades and FIU pond water, respectively. Methylation of inorganic mercury by CH 3 I in deionized water Experiments were conducted in deionized water, where factors (for example, DOM, Fe 2+ ) possibly facilitating the reduction of Hg 2+ are absent, to validate the aforementioned mechanism of photoinduced methylation of Hg 2+ by CH 3 I. The presence of CH 3 Hg + under sunlight was observed after 1 day of incubation when or Hg 0 was used as a precursor, while the methylation of Hg 2+ was not detected ( Supplementary Fig. 5 ). The formation of CH 3 Hg + was not observed for all three inorganic mercury precursors in the dark. These results demonstrate that Hg 2+ cannot be directly methylated by CH 3 I. In deionized water, the experimentally generated CH 3 Hg + became undetectable after 3 days ( Supplementary Fig. 5 ). This loss of CH 3 Hg + is not probably the results of photodegradation as previous studies showed that CH 3 Hg + present in deionized water cannot be photodemethylated [21] , [22] . During the course of the experiments, rapid degradation of CH 3 Hg + was always accompanied with a change in solution colour from clear to brown. The brown substance was identified to be I 2 based on the results of the following two experiments. A purple colour appeared in the organic phase when an extraction was performed with CH 2 Cl 2 (ref. 23 ), indicating this substance could be I 2 ( Supplementary Fig. 6 ). The brown solution turned blue when starch was added, indicating the formation of I 3 − amylose complex. Furthermore, ultraviolet-visible spectra analysis showed that the brown substance in water and the purple substance in CH 2 Cl 2 gave a maximum absorbance similar to that of I 3 − in water and I 2 in CH 2 Cl 2 , confirming the formation of I 2 ( Supplementary Fig. 6 ). I 2 may be produced from the combination of I·or through the oxidation of I − by dissolved oxygen (equations 6 and 7) [5] . Thus, it was assumed that I 2 , originating from CH 3 I, caused the degradation of CH 3 Hg + in deionized water. To test this hypothesis, I 2 or I − solution was added to deionized water containing . For trials with I 2 , immediate analysis of the solution indicated that disappeared completely ( Supplementary Fig. 7a ). An increase in the amount of 201 Hg 0 and 201 Hg 2+ was also observed, confirming the degradation of . However, the concentration of showed no significant change in the presence of I − ( Supplementary Fig. 7b ), indicating that I − could not degrade . In contrast to deionized water, the degradation of in natural water showed no significant difference ( P >0.1) in the presence or absence of CH 3 I ( Fig. 2 ). In addition, the water colour did not change to brown during the 5 days of incubation ( Supplementary Fig. 6 ). It is proposed that any I 2 formed would be quickly reduced to I − in the presence of humic substances [24] , thus inhibiting the degradation of CH 3 Hg + by I 2 . This assumption was partially supported by the fact that the rapid degradation of in the presence of CH 3 I was not observed when Suwannee River humic acid was added to deionized water ( Supplementary Fig. 8 ). The degradation of in Suwannee River humic acid solution correlated with cumulative photosynthetic active radiation (PAR) photon flux ( Supplementary Fig. 8 ), indicating that sunlight was the driver for the degradation of . The rapid degradation of CH 3 Hg + by I 2 would explain why the methylation of Hg 0 by CH 3 I was not detected under sunlight in deionized water in a previous study [11] . 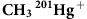Figure 2: Degradation ofin pond water. Solid line and dashed line represent the degradation of CH3Hg+in the presence (1 mmol l−1) or absence of CH3I, respectively. The degradation rate ofwas calculated to be 0.015±0.001 m2E−1in the presence of CH3I and 0.013±0.002 m2E−1without CH3I. The degradation of CH3Hg+showed no significant difference in the presence or absence of CH3I (P>0.1). All the tests were conducted in triplicate, and the error bars indicate the s.d. of three repeated measurements. Figure 2: Degradation of in pond water. Solid line and dashed line represent the degradation of CH 3 Hg + in the presence (1 mmol l −1 ) or absence of CH 3 I, respectively. The degradation rate of was calculated to be 0.015±0.001 m 2 E −1 in the presence of CH 3 I and 0.013±0.002 m 2 E −1 without CH 3 I. The degradation of CH 3 Hg + showed no significant difference in the presence or absence of CH 3 I ( P >0.1). All the tests were conducted in triplicate, and the error bars indicate the s.d. of three repeated measurements. Full size image Pathway of methylation of inorganic mercury by CH 3 I Based on the results obtained in deionized and natural waters, a pathway of photoinduced methylation of inorganic mercury by CH 3 I in natural water was proposed ( Fig. 3 ). Under the influence of solar irradiation, Hg 2+ can be reduced to Hg 0 or (probably facilitated by DOM) in natural waters [25] , while CH 3 I can be decomposed to CH 3 ·/I· or CH 3 + /I − . CH 3 · radicals and CH 3 + ions can then methylate or Hg 0 through oxidative addition reactions. DOM may play an important role in this process. On one hand, DOM can be an effective scavenger of I 2 , therefore inhibiting the degradation of CH 3 Hg + induced by I 2 . On the other hand, DOM may facilitate the reduction of Hg 2+ to Hg 0 or under sunlight [25] , subsequently enhancing the oxidative methyl transfer. 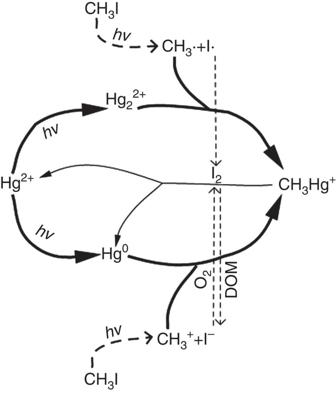Figure 3: Proposed pathway of photoinduced methylation of inorganic Hg by CH3I in natural water. The methylation of Hg by CH3I is proposed to include two steps, the reduction of Hg2+toor Hg0and the subsequent methylation ofor Hg0by CH3. or CH3+(solid line), which are photo-decomposition products of CH3I (dashed line). I2, which is produced from the combination of I· or oxidation of I−by dissolved oxygen, can rapidly degrade the generated CH3Hg+. However, this process is negligible in natural waters as I2can be quickly reduced to I−by DOM. Figure 3: Proposed pathway of photoinduced methylation of inorganic Hg by CH 3 I in natural water. The methylation of Hg by CH 3 I is proposed to include two steps, the reduction of Hg 2+ to or Hg 0 and the subsequent methylation of or Hg 0 by CH 3 . or CH 3 + (solid line), which are photo-decomposition products of CH 3 I (dashed line). I 2 , which is produced from the combination of I· or oxidation of I − by dissolved oxygen, can rapidly degrade the generated CH 3 Hg + . However, this process is negligible in natural waters as I 2 can be quickly reduced to I − by DOM. Full size image Assessment of CH 3 I-involved CH 3 Hg + formation in environments After being applied in farmland, CH 3 I could be transported into surrounding ponds or lakes via runoff water. The levels of CH 3 I in runoff water were estimated by laboratory column-leaching experiments ( Supplementary Fig. 9 ). CH 3 I applied to soils can be quickly leached out with concentration reaching 0.20–2.22 mmol l −1 depending on the soil type used ( Supplementary Fig. 9 ), which is two to five order of magnitude higher than its concentration in coastal waters [26] . The reaction of Hg 2+ and CH 3 I in pond water can be described as a pseudo-second-order reaction ( Fig. 4 ). The photomethylation rate constant of Hg 2+ by CH 3 I ( k M , see equation (13)) was then calculated to be (1.51±0.19) × 10 −2 l mol −1 E −1 m 2 in pond water. By using the obtained methylation rate constant and assuming that the increased CH 3 I concentration in aquatic water was in the range of 0–7 mmol l −1 (comparable to its concentration in leachates obtained in column experiments), the differences in CH 3 Hg + concentration at steady state in natural water with or without the presence of CH 3 I were estimated (equation (17)). Figure 5 showed that the increased steady-state concentration of CH 3 Hg + is highly dependent on the concentration of CH 3 I and Hg 2+ . 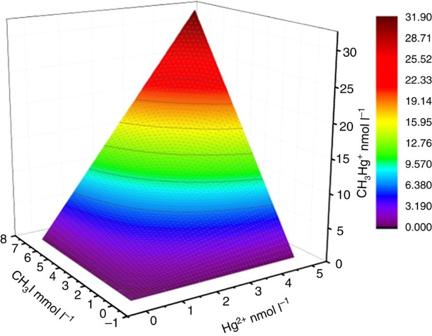Figure 5: The effects of CH3I and Hg2+on the increased steady-state concentration of CH3Hg+. The obtained photomethylation rate constant of Hg2+by CH3I (kM=1.51 × 10−2l mol−1E−1m2) and photodemethylation rate constant of CH3Hg+(kD=0.015 m2E−1) in the pond water were used to calculate the increased steady-state concentration of CH3Hg+(equation (17)). The concentrations of Hg2+and CH3I are assumed to be in the range of 0–5 nmol l−1and 0–7 mmol l−1, respectively. If we assume that the concentration of CH 3 I entering natural water is 1 mmol l −1 (comparable with that obtained in leachates) and Hg 2+ concentration is 6.1–3265.4 pmol l −1 (literature reported mercury levels in natural waters) [27] , [28] , the steady-state concentration of CH 3 Hg + in natural waters was estimated to increase by 0.005–2.966 pmol l −1 through the CH 3 I-involved methylation of mercury (see Supplementary Table 1 ). This increase in CH 3 Hg + is comparable to the concentration of CH 3 Hg + in these natural waters (<0.025–5.085 pmol l −1 ) [27] , [28] . To evaluate the relative importance of CH 3 I-involved methylation versus biotic methylation in sediments, we further compared the formation rate of CH 3 Hg + from photomethylation by CH 3 I in water body and the diffusion rate of CH 3 Hg + from sediment (generated by biotic methylation) with water (see Supplementary Table 2 ). The results showed that the calculated formation rates of CH 3 Hg + from photomethylation by CH 3 I are in the range of 0.53–258.5 pmol m −2 d −1 , comparable with the diffusion rates of CH 3 Hg + from sediment (−3.0–327.0 pmol m −2 d −1 ) ( Supplementary Table 2 ), indicating that CH 3 I-involved formation of CH 3 Hg + could be comparable with that diffused from sediment (mainly generated by biotic methylation). 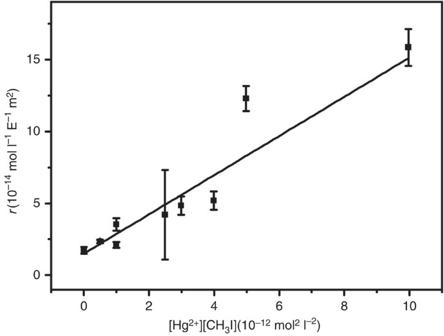Both estimations suggest that photomethylation of mercury by CH 3 I could be an important source of CH 3 Hg + in areas with CH 3 I fumigant application. Figure 4: Relationship between the formation rate of CH3Hg+and the product of Hg2+and CH3I concentrations in a pond water. To calculate the relationship between the formation rate of CH3Hg+(r) and concentrations of Hg2+and CH3I, various concentration of CH3I (0, 0.1, 0.2, 0.5, 1.0 and 2.0 mmol l−1) and199HgCl2(0, 1.0, 2.0, 3.0, 4.0 and 5.0 nmol l−1) were prepared using pond water containing 1 ng l−1(5.0 pmol l−1). The formation rate was observed to be positively related to the product of Hg2+and CH3I concentrations. Photomethylation rate constant of Hg2+by CH3I (kM, see equation (13) in main text) was calculated to be (1.51±0.19) × 10−2l mol−1E−1m2. All the tests were conducted in triplicate, and the error bars indicate the s.d. of three repeated measurements. Figure 4: Relationship between the formation rate of CH 3 Hg + and the product of Hg 2+ and CH 3 I concentrations in a pond water. To calculate the relationship between the formation rate of CH 3 Hg + ( r ) and concentrations of Hg 2+ and CH 3 I, various concentration of CH 3 I (0, 0.1, 0.2, 0.5, 1.0 and 2.0 mmol l −1 ) and 199 HgCl 2 (0, 1.0, 2.0, 3.0, 4.0 and 5.0 nmol l −1 ) were prepared using pond water containing 1 ng l −1 (5.0 pmol l −1 ) . The formation rate was observed to be positively related to the product of Hg 2+ and CH 3 I concentrations. Photomethylation rate constant of Hg 2+ by CH 3 I ( k M , see equation (13) in main text) was calculated to be (1.51±0.19) × 10 −2 l mol −1 E −1 m 2 . All the tests were conducted in triplicate, and the error bars indicate the s.d. of three repeated measurements. Full size image Figure 5: The effects of CH 3 I and Hg 2+ on the increased steady-state concentration of CH 3 Hg + . The obtained photomethylation rate constant of Hg 2+ by CH 3 I ( k M =1.51 × 10 −2 l mol −1 E −1 m 2 ) and photodemethylation rate constant of CH 3 Hg + ( k D =0.015 m 2 E −1 ) in the pond water were used to calculate the increased steady-state concentration of CH 3 Hg + (equation (17)). The concentrations of Hg 2+ and CH 3 I are assumed to be in the range of 0–5 nmol l −1 and 0–7 mmol l −1 , respectively. Full size image Methylation of mercury by sulphate-reducing [29] or iron-reducing bacteria [30] has been deemed to be the main source of CH 3 Hg + in aquatic environments. However, this study shows that methylation of inorganic mercury by CH 3 I could be another important source of CH 3 Hg + . This would be particularly true in an environment where CH 3 I is used in large amounts as a fumigant. In addition to acting as a methylation agent, CH 3 I can also serve as a potential mobilizing agent for mercury sulfide (HgS) [12] . It has been demonstrated that CH 3 I could methylate sulphide into volatile (CH 3 ) 2 S and (CH 3 ) 2 S 2 , and then liberate free Hg 2+ into water from insoluble HgS [12] . Considering HgS is an important inorganic mercury species in anoxic environments such as soil [31] , sediment [32] and sulphidic water [33] , this dissolution process of HgS could increase the leaching and release of Hg 2+ from soil and sediment into surface water, and therefore enhance the potential formation of CH 3 Hg + . As CH 3 Hg + is a neurotoxin, the impact of CH 3 I application to farmland on biogeochemical cycling of mercury should be carefully evaluated. With respect to the production of CH 3 Hg + , most previous studies focused on the methylation of Hg 2+ in the environment; however, there is a lack of knowledge on the methylation of Hg 0 . Results of this study imply that methylation of Hg 0 can occur in the environment (for example, by CH 3 I). Although Hg 0 is present at low concentrations in water and sediment, Hg 2+ , through photomediated reduction in natural waters, provides a sufficient and continuous source of Hg 0 . Additionally, Hg 0 is the main Hg species in the atmosphere, and the co-occurrence of Hg 0 and released CH 3 I from fumigated fields by volatilization, makes the photochemical methylation of Hg 0 possible in the atmosphere. Therefore, the methylation of Hg 0 by CH 3 I and its contribution to the CH 3 Hg + pool needs to be considered. Fumigants are widely applied in agricultural fields to control pests and weeds. With the phase out of CH 3 Br, the use of CH 3 I is expected to increase dramatically in the future. CH 3 I is a pulmonary and dermal irritant [26] , and is also suspected to be carcinogenic [34] , neurotoxic [18] , [26] and endocrine disrupting [4] . This study shows that CH 3 I could also indirectly threaten the health of humans and wildlife by forming a toxic chemical, CH 3 Hg + , suggesting the necessity of a more comprehensive risk assessment of CH 3 I use as a fumigant. In summary, we have demonstrated that the registered fumigant CH 3 I could methylate inorganic Hg species, including Hg 0 , and Hg 2+ , into toxic CH 3 Hg + in natural water under sunlight. The photoinduced CH 3 Hg + formation mechanism by CH 3 I is proposed, which involves the reduction of Hg 2+ to Hg 0 / and the subsequent methylation of Hg 0 / by CH 3 I, following an oxidative addition reaction. Quantitative assessment suggests that methylation of inorganic Hg by CH 3 I could be an important source of CH 3 Hg + in CH 3 I-contaminated surface water. Reagents CH 3 Hg + standard was purchased from Ultra Scientific (North Kingstown, RI). Enriched 201 HgO and 199 HgO were purchased from Oak Ridge National Laboratory (Oak Ridge, TN). was synthesized from enriched 201 HgO using methylcobalamin [35] . Enriched 199 HgCl 2 solution was prepared by dissolving 199 HgO in 10% HCl. Elemental mercury (Hg 0 ) and Hg 2 (NO 3 ) 2 were purchased from Fisher Chemicals (Pittsburgh, PA). Hg 0 stock solution was freshly prepared following the method by Whalin and Mason [36] . One drop of Hg 0 was first transferred into a piece of silicon tubing. After capping at both ends with Teflon plugs, the tubing was immersed into deionized water. Next, the gaseous Hg 0 was equilibrated with water for over 48 h under anoxic conditions. The concentration of Hg 0 in water was determined before the experiment was conducted. CH 3 I and CD 3 I were purchased from Fisher Chemicals and Hengye Zhongyuan Chemicals (Beijing, China), respectively. Deionized water was prepared from a Barnstead NANOpure Diamond Life Science (UV/UF) ultrapure water system (Barnstead International, Dubuque, IA). Methylation of inorganic mercury by CH 3 I Water samples were collected from a pond in FIU (25°45′N, 80°22′W) and the Florida Everglades (25°45′N, 80°44′W), and stored in pre-cleaned 2-L Teflon bottles using trace metal clean procedures. The samples were kept in a cooler and transported to the laboratory within 3 h. Methylation experiments were conducted immediately on arrival at the laboratory. The methylation experiments were carried out in a 0.5-l Teflon bottle under natural sunlight or in darkness (wrapping bottles with aluminum foil). 199 HgCl 2 , Hg 2 (NO 3 ) 2 or Hg 0 was spiked into each bottle to form a final concentration of about 1,000 ng l −1 (4.99 nmol l −1 ) as mercury, respectively. CH 3 I and CH 3 201 Hg were then added to each bottle to form a final concentration of 141.9 mg l −1 (1 mmol l −1 ) and 1 ng l −1 (4.975 pmol l −1 ), separately. For the experiments conducted in deionized water, 199 HgCl 2 , Hg 2 (NO 3 ) 2 or Hg 0 was spiked to each bottle to form a final concentration of about 1,000 ng l −1 (4.99 nmol l −1 ) as mercury, respectively. CH 3 I were then added to each bottle to form a final concentration of 141.9 mg l −1 (1 mmol l −1 ). To investigate the effects of Hg 2+ and CH 3 I concentrations on the methylation rate, various concentration of CH 3 I (0, 0.1, 0.2, 0.5, 1.0 and 2.0 mmol l −1 ) and 199 HgCl 2 (0, 1.0, 2.0, 3.0, 4.0 and 5.0 nmol l −1 ) were spiked into pond water containing 4.99 pmol l −1 . Bottles were incubated under ambient temperature and light conditions for 4 days. During the experiment, the intensity of ambient PAR was measured at 15min intervals routinely using LI-192 Quantum Sensor (LI-COR Biosciences, Lincoln, NE). Triplicates (three separate bottles) were employed for each trial. CH 3 202 Hg + , and CH 3 199 Hg + in the incubated samples were determined after 0, 0.5, 1, 2, 3 and 4 days of incubation using the aqueous phenylation purge-and-trap followed by the GC inductively coupled plasma–MS (ICP-MS) detection. A CD 3 I addition technique was adopted to investigate the origin of the methyl group in the generated CH 3 Hg + . HgCl 2 and CD 3 I were added to 2 l of environmental water to form a final concentration of 9.97 μmol l −1 as Hg 2+ and 20 mmol l −1 , respectively. The bottle was then incubated under ambient temperature and light conditions for 4 days. The formation of CD 3 Hg + was verified by the aqueous phenylation–solid phase microextraction (SPME)–GC–MS. Analysis of CH 3 Hg + Water samples (20 ml), L -ascorbic acid (100 mmol l −1 , 1 ml), concentrated HCl (1 ml) and CH 2 Cl 2 (5 ml) were added into a 50-ml polypropylene centrifuge tube (Corning Inc, Lowell, MA) sequentially. After shaking for 30 min, the samples were left to stand for 5 min to let CH 2 Cl 2 separate from water. CH 2 Cl 2 (2.5 ml) phase was then transferred to a 50-ml polypropylene centrifuge tube containing 35 ml 1% (v/v) HCl. The tube was purged with N 2 at 150 ml min −1 to completely volatilize CH 2 Cl 2 and release CH 3 Hg + into aqueous phase. CH 3 Hg + in the aqueous phase was analysed by aqueous phenylation and purge-and-trap pre-concentration followed by GC–ICP–MS [37] . The artificial formation of CH 3 Hg + using this method has been demonstrated to be negligible, attributing to the omission of the distillation procedure and the replacement of the derivatization reagents (from sodium tetraethylborate or sodium (n-propyl)borate to sodium phenylborate (NaBPh 4 )) [37] . Aqueous phenylation reactions were performed in 300-ml glass bubblers from Exeter Scientific Glass Co. (Birdsboro, PA). The prepared sample (35 ml) was added to a 100 ml solution containing 30% (w/v) NaCl and 0.17% (w/v) NaOH. Two millilitres of citric buffer (pH 5.0, 2 mol l −1 ) and 1 ml of 1% (w/v) NaBPh 4 (Fisher Chemicals, Fairlawn, NJ) were added. After 15 min of reaction, the phenylation products were purged from the bubbler at 45 °C for 45 min with 200 ml min −1 of N 2 , and trapped on a Tenax trap. The trap was dried for 5 min by 200 ml min −1 of N 2 . Finally, the trapped mercury species were thermally desorbed and separated using a fused silica capillary column (15 m × 0.53 mm i.d., coated with DB-1 film of 1.5-μm thickness) and then measured with an Elan DRC-e ICP-MS (PerkinElmer Sciex, Waltham, MA). Phenylation–SPME–GC–MS [38] was used to validate the origin of the methyl group in produced CH 3 Hg + . Natural waters (2,000 ml) were transferred to 2-l Teflon bottles and spiked with 4 mg Hg 2+ and 40 mmol CD 3 I. The solution was incubated under ambient temperature and sunlight for 4 days. The produced CD 3 Hg + was extracted from each 40-ml water sample after adding 1 ml concentrated HCl and 5 ml CH 2 Cl 2 . The CH 2 Cl 2 phase (4 ml) was transferred into a 100-ml polypropylene centrifuge tube containing 35 ml 1% HCl and purged with N 2 at 150 ml min −1 to remove CH 2 Cl 2 . Then, pH was adjusted to 7 using 0.17% (w/v) NaOH. Sample solution (35 ml), 2 mol l −1 HAc-NaAc buffer (5 ml, pH 4.9) and 15 g NaCl were added to a 100-ml glass vial sealed with a polytetrafluoroethylene-coated septum. One millilitre 1% (w/v) NaBPh 4 solution was injected into the vial using a syringe. The vial was stirred by a magnetic stirring bar and maintained at 55 °C for 30 min in an oven. Next, headspace SPME extraction was carried out at 55 °C for 10 min. After extraction, the fibre was introduced into the GC injection port (200 °C) for thermal desorption and GC–MS analysis in splitless mode. The GC temperature programming is as following: 80 °C for l min, increased to 280 °C at a rate of 8 °C min −1 and held there for 10 min. Analysis of Hg 0 Hg 0 in water was purged and trapped onto a home-made gold trap and detected by atomic fluorescence spectrometer. Hg 2+ solution was used as the calibration standard. Hg 2+ standard and 0.5 ml SnCl 2 solution (10% (w/v)) were added to 100 ml 1% (v/v) HCl. The mixture was left to react for 15 min and then purged for 20 min with 400 ml min −1 of N 2 at room temperature to let Hg 0 completely volatilize and adsorb on the gold trap. The trap was dried for 5 min by 400 ml min −1 of N 2 . Finally, the trapped Hg 0 was thermally desorbed and determined by a PS Analytical mercury speciation system (Orpington, Kent, UK). The analytical procedure for purgeable Hg 0 in water samples was similar to that for the Hg 2+ standards, except that SnCl 2 and HCl were not added. Characterization of using Raman spectrometry Formation of during the photoreduction of Hg 2+ was investigated using surface-enhanced Raman spectrometry. Suwannee River humic acid and Hg 2+ were added into deionized water to form a final concentration of 40 mg l −1 dissolved organic carbon and 0.5 mmol l −1 Hg 2+ , respectively. After incubation under sunlight for 3 days, Raman-scattering spectra of in the solution with and without the addition of KI (1.0 mol l −1 ) were collected using the following method. Au nanoparticle (AuNPs) solution was prepared by heating the solution containing 1 mol l −1 AuCl 4 − and 5 mg l −1 dissolved organic matter (pH 6.8) at 80 °C for 24 h [39] . AuNP-coated Si wafer was then made by dropping AuNPs on Si wafer and then dried in a vacuum desiccator at room temperature. Next, water samples containing mercury species were dropped on the wafer and dried in a vacuum desiccator at room temperature. The AuNPs-enhanced Raman-scattering spectra of samples were obtained by using a Leica microscope in a confocal Raman spectroscopy system (Renishaw InVia Raman microscope, Britain). Spectra collections were carried out using a × 50 objective lens and 60-s scan between 155.48 and 1,132.18 cm −1 with a 532-nm laser (5 mW) and 2,400 lines per mm grating. Column experiments for evaluating the leachability of CH 3 I The leachability of CH 3 I was investigated using columns (16 cm length × 5 cm i.d.) containing vegetable soil, sandy soil or quartz sand. To minimize the losses of soil during the experiment, a well-permeable quartz plate was placed at the bottom of the column and the top 3 cm of the columns was filled with quartz sand. The columns were pre-saturated with deionized water and then 27.36 mg CH 3 I (corresponding to an application rate of 125 lb ac −1 ) was added into the columns. The columns were then leached with deionized water at a rate of 4.1 ml min −1 for 3 h. Leachates (50 ml) were continuously collected at an interval of ~12 min. Leachates (10 ml) in 15-ml polypropylene centrifuge tube were extracted with CH 2 Cl 2 (2 ml) (Corning Inc, Lowell, MA). After shaking for 30 min, the samples were left to stand for 5 min to let CH 2 Cl 2 separate from water. One ml CH 2 Cl 2 phase was collected for GC–MS analysis. The determination of CH 3 I was performed using an Agilent 7,890 gas chromatograph system, coupled to a quadruple Agilent 5,975 electron ionization mass spectrometric detector (Agilent Technologies, Palo Alto, CA, USA) equipped with a DB-624 fused silica capillary column (30 m × 0.25 mm i.d., 1.4-μm film thickness). The gas chromatograph system was equipped with a split/splitless injection port operating in split mode (50:1) at 120 °C. The injection volume was 2 μl. The oven temperature was programmed from 40 °C (2 min) to 90 °C at 5 °C min −1 , and then to 240 °C at 15 °C min −1 . The carrier gas was helium with a constant flow of 1 ml min −1 . The mass spectrometer was operated in SIM mode ( m/z =127 and 142). Solvent delay was set at 2 min. Quantification was conducted using an external standard curve method. Data analysis The methylation rates of Hg 0 , and Hg 2+ ( r ) were calculated by nonlinear regression of CH 3 Hg + concentration against t using equation (9) (Origin, Version 6.0 for Windows, OriginLab Corp., Northampton, MA). The net production rate of CH 3 Hg + can be described as the difference of the photomethylation rate of inorganic mercury by CH 3 I ( r × PAR ) and the photodegradation rate of CH 3 Hg + ( ) at t time (equation (8)). Next, the function of at t time could be obtained (equation (9)) by integrating equation (8). Degradation of CH 3 Hg + can occur in natural waters and this process was deemed to be driven by sunlight [21] , [40] . In this study, the spiked was also observed to be rapidly degraded under sunlight in both tested waters, while degradation of was not observed in the dark. The effect of CH 3 Hg + photodegradation was taken into account in the calculation, represented by the photodegradation rate constant k D . A model based on the first-order chemical kinetics was used to describe the photodegradation of in water (equation (10)) [21] , [40] . The rate constant of photodegradation, k D , was calculated by linear regression of against t . where and are the concentrations of CH 3 Hg + at the beginning and t time, respectively (pmol l −1 ), k D is the rate constant of CH 3 Hg + photodegradation (m 2 E −1 ), PAR is the photosynthetically active radiation (E m −2 d −1 ), J is the cumulative PAR photon flux (E m −2 ) and r is the PAR normalized formation rate of CH 3 Hg + (pmol l −1 E −1 m 2 ). The differences in CH 3 Hg + concentrations at steady state with or without the presence of CH 3 I were calculated and used to evaluate the influence of CH 3 I on CH 3 Hg + production. In natural waters, the concentration of CH 3 Hg + was assumed to be determined by several key processes, including photodegradation of CH 3 Hg + , input of CH 3 Hg + from sediment and runoff, methylation in water body and methylation by CH 3 I. Next, the changing rate of CH 3 Hg + could be calculated by the photodegradation rate , the CH 3 Hg + input rate from sediment and runoff ( R 0 ), the methylation rate ( R ′) and the rate of photomethylation by CH 3 I ( r × PAR ). As r was found to be positively related to the product of and (equation (13), Fig. 4 ) and equation (14) could be obtained by combining equation (13) with equation (12). where R 0 is the rate of CH 3 Hg + input from sediment and runoff (pmol l −1 d −1 ), R ′ is the non-CH 3 I involved methylation rate in water body (pmol l −1 d −1 ), k M is the PAR -normalized formation rate constant of CH 3 Hg + (l pmol −1 E −1 m 2 ), is the concentration of Hg 2+ (pmol l −1 ), is the concentration of CH 3 I (pmol l −1 ). The predicted concentration of CH 3 Hg + at steady state in the presence of CH 3 I ( ) can be calculated by making the right side of equation (14) equal to zero (equation (15)). The predicted concentration of CH 3 Hg + at steady state in the absence of CH 3 I ( ) can be calculated by making of equation (15) equal to zero (equation (16)). Next, the differences in CH 3 Hg + concentrations at steady state with or without the presence of CH 3 I ( ) can be calculated by equation (17). The parameters for calculating are given in Supplementary Table 1 . To evaluate the relative importance of CH 3 I-involved methylation versus biotic methylation, the CH 3 Hg + photomethylation rate within the entire water column was calculated as follows. The sunlight intensity at Z depth (m) is calculated from the light intensity in the surface water ( PAR (0)) by exponentially decreasing it with depth according to the Beer-Lambert equation. Combined with the calculation of the photomethylation rate of CH 3 Hg + in the surface water, the photomethylation rate at Z depth can be described as equation (18). Next, mercury methylation is integrated with respect to water column depth to obtain the methylation rate within the entire water column (equation (19)). where is the concentration of CH 3 Hg + at depth Z (pmol l −1 ), PAR (0) is the PAR above the surface of the water (E m −2 d −1 ) and k is the light attenuation coefficient of sunlight (m −1 ). Then, The parameters for calculating are given in Supplementary Table 2 . How to cite this article: Yin, Y. et al . Fumigant methyl iodide can methylate inorganic mercury species in natural waters. Nat. Commun. 5:4633 doi: 10.1038/ncomms5633 (2014).